Trends in the development of environmentally friendly fouling-resistant marine coatings 'arine biofouling, the colonization of submerged surfaces by unwanted marine organisms ( Fig. 1 ), has detrimental effects on shipping and leisure vessels, heat exchangers, oceanographic sensors and aquaculture systems. For example, it has been shown that the increased roughness presented by a heavily fouled ship hull can result in powering penalties of up to 86% at cruising speed; even relatively light fouling by diatom 'slimes' can generate a 10–16% penalty [1] . Without effective antifouling (AF) measures, in order to maintain speed, fuel consumption (and therefore greenhouse gas emissions [2] ) increase significantly. A recent analysis of the economic impact of biofouling for the Arleigh Burke DDG-51 destroyers, which comprise 30% of the ships in the US Navy fleet, estimates the overall cost associated with hull fouling at $56 million per annum [3] . This figure is based on the present AF coating system, cleaning and fouling level (typically heavy slime) of the Navy. If the analysis is extended to the entire US Navy fleet, the approximate cost of hull fouling is between $180 and 260 million per annum. 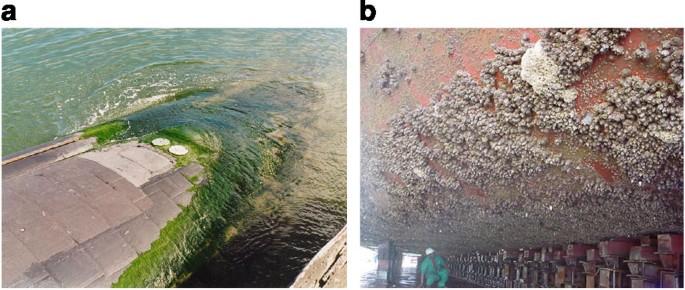Figure 1: Vessels fouled by marine organisms. Images show (a) fouling by the green alga (seaweed)Ulva(image courtesy of Dr J. Lewis) and (b) barnacles (image courtesy of Dr C.D. Anderson). Figure 1: Vessels fouled by marine organisms. Images show ( a ) fouling by the green alga (seaweed) Ulva (image courtesy of Dr J. Lewis) and ( b ) barnacles (image courtesy of Dr C.D. Anderson). Full size image Marine biofouling is ubiquitous and has been a practical problem ever since man sailed the oceans; controlling it, without simultaneously creating unacceptable environmental impacts on non-target species is a considerable challenge. Recent years have seen a resurgence of interest in the fundamental science behind the processes involved in biofouling, and in the design of novel coatings and other non-coating technologies. The main driver for this is legislation that has outlawed some highly effective AF paints, notably the use of tributyltin oxide, and posed a stricter evaluation and regulatory regime on the use of alternative biocides. 'Green' alternatives to biocide-based technologies are therefore urgently sought by the marine coatings industry, and there is considerable interest in developing biocide-free coatings that rely on surface physico-chemical and bulk materials properties to either deter organisms from attaching in the first place ('prevention is better than cure') or reduce the adhesion strength of those that do attach, so that they are easily removed by the shear forces generated by ship movement or mild mechanical cleaning devices. Fouling-resistant coatings for application to large-scale structures, such as ship hulls, are based on polymeric 'binders'—the film-forming component of paint. Advances in macromolecular synthesis, self-assembling polymers, hyperbranched and interpenetrating polymer networks and various types of nanocomposites, provide opportunities for developing novel binder systems. Natural AF surfaces also provide a source of inspiration for new coating designs. This review is aimed at the intersection between biology, materials sciences and engineering. Biological aspects of fouling and the particular challenges posed to the materials scientist confronted by the vast biodiversity in fouling species and the range of attachment behaviours and adhesion mechanisms adopted will first be considered. Some of the novel approaches currently being explored by materials scientists in developing coatings for marine applications, both from a fundamental and more practical perspective, will then be discussed. Emphasis will be given to interdisciplinary studies in which the structure and surface properties of coatings are correlated with their biological performance or in which predictive models are being developed that will facilitate rational design of coatings in the future. When a clean surface is immersed in natural seawater, it immediately starts to adsorb a molecular 'conditioning' film primarily consisting of dissolved organic material [4] . Colonization of the conditioned surface by a wide range of organisms depends on the availability of the colonizing stages, and their relative rates of attachment and surface exploitation. Fouling is a highly dynamic process; the specific organisms that develop in a fouling community depend on the substratum, geographical location, the season and factors such as competition and predation. A distinction is often made among 'microfouling' (often referred to as 'slime') due to unicellular microorganisms such as bacteria, diatoms and protozoa, which form a complex biofilm; 'soft macrofouling' comprising macroscopically visible algae (seaweeds) and invertebrates such as soft corals, sponges, anemones, tunicates and hydroids; and 'hard macrofouling' from shelled invertebrates such as barnacles, mussels and tubeworms ( Fig. 2 ). 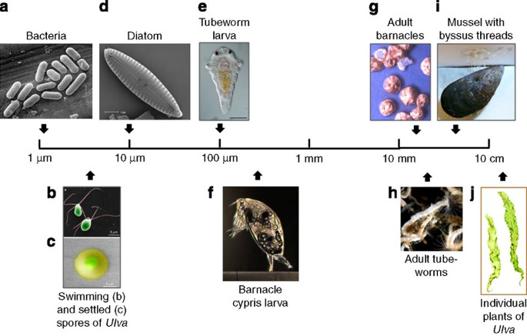Figure 2: Diversity and size scales of a range of representative fouling organisms. (a) Bacteria (scanning electron micrograph (SEM)), (b) false-colour SEM of motile, quadriflagellate spores of the green alga (seaweed)Ulva, (c) false-colour environmental SEM image of settled spore ofUlvashowing secreted annulus of swollen adhesive, (d) SEM of diatom (Navicula), (e) larva of tube worm,Hydroides elegans(image courtesy of B. Nedved), (f) barnacle cypris larva (Amphibalanus amphitrite) exploring a surface by its paired antennules (image courtesy of N. Aldred), (g) adult barnacles (image courtesy of AS Clare), (h) adult tubeworms (H. elegans; image courtesy of M. Hadfield), (i) adult mussels showing byssus threads attached to a surface (image courtesy of J. Wilker), (j) individual plants of the green alga (seaweed)Ulva. The diagram is intended to indicate relative scales rather than absolute sizes; individual species within a group can vary significantly in absolute size. Figure 2: Diversity and size scales of a range of representative fouling organisms. ( a ) Bacteria (scanning electron micrograph (SEM)), ( b ) false-colour SEM of motile, quadriflagellate spores of the green alga (seaweed) Ulva , ( c ) false-colour environmental SEM image of settled spore of Ulva showing secreted annulus of swollen adhesive, ( d ) SEM of diatom ( Navicula ), ( e ) larva of tube worm, Hydroides elegans (image courtesy of B. Nedved), ( f ) barnacle cypris larva ( Amphibalanus amphitrite ) exploring a surface by its paired antennules (image courtesy of N. Aldred), ( g ) adult barnacles (image courtesy of AS Clare), ( h ) adult tubeworms ( H. elegans ; image courtesy of M. Hadfield), ( i ) adult mussels showing byssus threads attached to a surface (image courtesy of J. Wilker), ( j ) individual plants of the green alga (seaweed) Ulva . The diagram is intended to indicate relative scales rather than absolute sizes; individual species within a group can vary significantly in absolute size. Full size image It is often stated that surface colonization follows a linear 'successional' model [5] , [6] , [7] , [8] , [9] in which bacterial biofilm formation is followed within a week by spores of macroalgae (seaweeds), fungi and protozoa, followed in turn, within several weeks, by larvae of invertebrates, such as barnacles. In reality, this 'classical' view is a considerable oversimplification as motile spores of seaweeds are capable of settling within minutes of presenting a clean surface [10] and larvae of some species of barnacles, bryozoans and hydroids settle within a few hours of immersion [11] . For both algae and larvae, this is well within the 'one-to-several weeks' quoted by Wahl [6] . Rather than the linear successional model, the 'dynamic' model [12] , [13] provides a more balanced view. It is also misleading to assume that successional colonization of a surface necessarily implies a causal relationship between one stage and the next and even more misleading to assume that controlling or blocking initial stages of colonization, such as biofilm formation, will reduce or eliminate macrofouling. On the other hand, it is undoubtedly clear that attachment of spores and larvae can be influenced by other organisms, notably by bacterial biofilms, and positive, negative and neutral effects have been detected in controlled laboratory experiments when biofilms of specific bacteria have been tested against algal spores and larvae of invertebrates [14] , [15] , [16] , [17] , [18] . Some of these effects have also been reported in field observations [16] . However, colonization models are mostly based on studies of natural substrata, such as wood and stone or traditional AF coatings that rapidly foul, and there are only a few reports that study the colonization of modern, non-biocidal AF coatings by microorganisms [19] , [20] . Fouling by biofilms composed of communities of bacteria, diatoms, fungi and protozoa has been largely ignored until recently, because the focus of research has been on macrofouling. It is likely that more attention will be paid to slime fouling in future, now that its economic impact is firmly established [1] , [3] . A major challenge in creating an effective fouling-resistant coating is that the diversity of fouling organisms is vast and the range of adhesion mechanisms (including adhesives) used is correspondingly great ( Fig. 2 ). The colonizing ('recruitment') stages of fouling organisms range in size from micrometres (bacteria, single-celled spores of algae and some diatom cells) to hundreds of micrometres or even millimetres (larvae of invertebrates). Considerations of size are relevant to attempts (see Future Directions ) to engineer surface topographies that may deter the settlement of organisms. However, the critical length scale in determining settlement is not necessarily the size of the organism per se , but rather the size of the parts or structures involved in the sensing apparatus of an organism (for example, the paired sensory antennules of barnacle cypris larvae [21] ( Fig. 2 )), which determine whether the organism selects a surface for attachment. Assuming that the organism has settled, the success of that organism in colonizing a surface and growing into a reproductive adult, within a turbulent marine environment, depends on how well the macromolecular adhesive polymers secreted by the settled organisms secure to the adhesive interface, which is determined by the interfacial molecular interactions that are in turn influenced by the properties of a surface or coating at the molecular or nanoscale level. Non-biocidal, fouling-resistant coatings are based on polymers designed to minimize molecular adhesive forces between the adhesives used by marine organisms and the coating. Rational design of coatings ultimately requires an elucidation of the chemical and physical interactions between the bioadhesives used by marine organisms and the prospective fouling-release polymer(s). Unfortunately, so few marine bioadhesives have been isolated and characterized that obtaining information at this level has proved to be difficult (see ref. 22 for comprehensive reviews of bioadhesives). An exception to this is the well-characterized marine mussel foot adhesive system based on byssal threads and adhesive plaques formed from a composite of several proteins [23] . Catechol groups of the amino acid DOPA (dihydroxyphenylalanine) are oxidized to react with other catechol groups to crosslink the proteins into a strong cohesive composite. Dihydroxyphenylalanine groups also hydrogen bond to metal ions in the mineral substrata. Surface-sensitive spectroscopic techniques have been used to understand molecular interactions between mussel adhesive proteins and various interfaces in situ . For example, sum frequency generation vibrational spectroscopy (SFG) has shown how substrate surface chemistry influences the structure of the adsorbed adhesive plaque protein Mefp-3 [24] . On a hydrophobic, non-polar substrate, to which Mefp-3 attaches weakly, strong SFG signals were detected in both C–H stretching and amide I regions, indicating that the adsorbed protein was in an ordered conformation. On a polar, hydrophilic polymer substrate to which Mefp-3 strongly adheres, no SFG signals in these regions were detected, showing that the protein adopted a more or less random or disordered structure. Application of this type of analysis to films based on polymers used in fouling-release coatings will prove instructive; however, until more marine adhesives of important fouling organisms are biochemically characterized and made available in purified form and in sufficient quantity for experimental purposes, the biophysical analysis of molecular events at adhesive/coating interfaces will have only limited impact on the design of novel coatings. One approach to the development of novel AF coatings is to create a 'deterrent' surface that inhibits the initial attachment of the recruitment ('settling') stages of spores, larvae and so on. These settling stages are 'choosy' in the sense that they exhibit behaviours that result in a surface being accepted or rejected for settlement. Although much can be done to assess such behavioural traits through simple assays of the ability of larvae or spores to settle on a surface, a more comprehensive understanding requires detailed observation of the behaviour of organisms as they explore the interface. In this section, we outline two current imaging technologies that are being used to enhance our understanding of organism behaviour in relation to specific surface properties. This information will provide improved insight into the chemistry and thermodynamics of adhesion and will help to formulate the 'design rules' by which novel materials may be developed to deter settlement. Two-dimensional tracking of the cypris larvae of barnacles has been studied using EthoVision tracking software [25] . Aldred et al . [26] explored cyprid behaviour on two zwitterionic polymer coatings (poly(sulfobetaine methacrylate) (polySBMA) and poly(carboxybetaine methacrylate) (polyCBMA)), both of which completely inhibited cyprid settlement and are resistant to protein adsorption [27] . On polySBMA and on bare glass, cyprids explored the surface, but were unwilling or unable to settle ( Fig. 3 ), whereas on polyCBMA, cyprids did not attempt exploration and left the surface quickly. 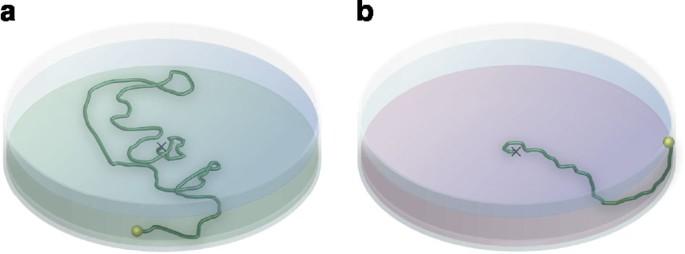Figure 3: Representative tracking patterns of barnacle cypris larvae exploring two zwitterionic surfaces. The motile cypris larvae of barnacles are 'choosy', that is, they explore the suitability of a surface for eventual adhesion by swimming over it, making 'sampling' contacts. The cartoon illustrates an experiment in which the bottom surface of two transparent dishes was coated with either (a) poly(sulfobetainemethacrylate) (polySBMA) or (b) poly(carboxybetainemethacrylate) (polyCBMA). (Note: The two coatings are actually colourless, but are shown as different colours to aid understanding). The dishes were filled with seawater before introducing the barnacle cypris larvae. The green lines illustrate the representative tracks of an individual larva on each surface, starting at or near the centre of the dish. Behaviour on polySBMA (a) is characterized by broad, sweeping deviations in the recorded track, with occasional contacts with the surface and abrupt changes in direction. This behavior suggests that the larvae are actively exploring this surface. Behaviour on polyCBMA (b) is quite different. Here, the larvae spent little time either swimming over the surface or making contacts with it, swimming immediately to the edge of the dish. Cartoon represents original data in ref.26. Figure 3: Representative tracking patterns of barnacle cypris larvae exploring two zwitterionic surfaces. The motile cypris larvae of barnacles are 'choosy', that is, they explore the suitability of a surface for eventual adhesion by swimming over it, making 'sampling' contacts. The cartoon illustrates an experiment in which the bottom surface of two transparent dishes was coated with either ( a ) poly(sulfobetainemethacrylate) (polySBMA) or ( b ) poly(carboxybetainemethacrylate) (polyCBMA). ( Note : The two coatings are actually colourless, but are shown as different colours to aid understanding). The dishes were filled with seawater before introducing the barnacle cypris larvae. The green lines illustrate the representative tracks of an individual larva on each surface, starting at or near the centre of the dish. Behaviour on polySBMA ( a ) is characterized by broad, sweeping deviations in the recorded track, with occasional contacts with the surface and abrupt changes in direction. This behavior suggests that the larvae are actively exploring this surface. Behaviour on polyCBMA ( b ) is quite different. Here, the larvae spent little time either swimming over the surface or making contacts with it, swimming immediately to the edge of the dish. Cartoon represents original data in ref. 26 . Full size image Although tracking the behaviour of fouling organisms aids in understanding surface selection, a more detailed understanding of interfacial interactions also requires information at the molecular level. Imaging surface plasmon resonance (iSPR) has been applied to in situ , real-time analysis of temporary adhesive deposition by barnacle larvae as they explore a surface [28] . Footprints of temporary adhesive were imaged on a bare gold-coated surface and a self-assembled monolayer of oliogoethylene glycol, selected for its well-known resistance to protein adsorption. Larvae were observed to probe both surfaces with their sensory structures, but only on the bare gold surface did the point of contacts leave deposits of temporary adhesive ( Fig. 4 ). The frequency with which the secreted protein sticks to the surface provides a proxy indication of the strength of the protein-surface bond [28] . This example demonstrates the power of iSPR to generate novel information on the exploration of different surfaces at the molecular level; what is now needed is to apply this approach to more complex, candidate experimental coatings for marine application, rather than simple model substrates, such as OEGs (oligo(ethyleneglycol))—this may require further technical improvements to iSPR. 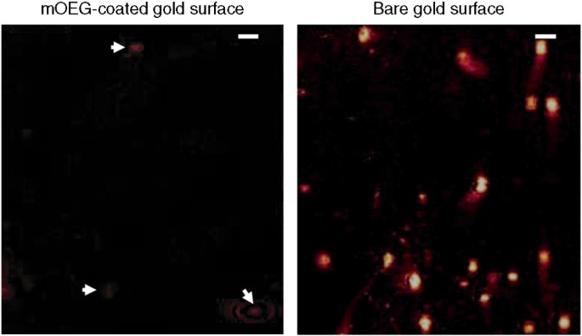Figure 4: Deposition of 'footprints' of the temporary protein adhesive secreted by cypris larvae of barnacles during surface exploration as revealed by imaging surface plasmon resonance. SPR is a spectroscopic, surface analysis technique that allows the adsorption of macromolecules to a metallic surface to be measured and imaged through changes in reflectivity. The two panels show snapshots of gold surfaces after cypris larvae were allowed to explore for 7 min. One of the gold surfaces was coated with methyl-terminated oligo(ethyleneglycol) (mOEG), the other was left as bare gold. On the bare gold surface, the cyprids explored the surface via their sensory antennules and made numerous contact points or 'footprints', shown as bright reflective spots, each of which represents the deposition of small amounts of proteinaceous temporary adhesive from the antennules. On the gold surface, these spots persisted following detachment of the cyprid, implying that the adhesive remained on the surface. In the case of the mOEG substrate, which is well known for its protein-repellent properties, although the cyprids explored the surface, very little proteinaceous residue remains at the contact points, as shown by the few, dull-reflective spots (arrowed). On mOEG, the spots only persisted for as long as the cyprid remained in contact with the surface implying that, on detachment, the protein remained on the antennules. The scale bars in each frame are 100 μm. Reproduced with permission from ref.28, © 2008 American Vacuum Society. Figure 4: Deposition of 'footprints' of the temporary protein adhesive secreted by cypris larvae of barnacles during surface exploration as revealed by imaging surface plasmon resonance. SPR is a spectroscopic, surface analysis technique that allows the adsorption of macromolecules to a metallic surface to be measured and imaged through changes in reflectivity. The two panels show snapshots of gold surfaces after cypris larvae were allowed to explore for 7 min. One of the gold surfaces was coated with methyl-terminated oligo(ethyleneglycol) (mOEG), the other was left as bare gold. On the bare gold surface, the cyprids explored the surface via their sensory antennules and made numerous contact points or 'footprints', shown as bright reflective spots, each of which represents the deposition of small amounts of proteinaceous temporary adhesive from the antennules. On the gold surface, these spots persisted following detachment of the cyprid, implying that the adhesive remained on the surface. In the case of the mOEG substrate, which is well known for its protein-repellent properties, although the cyprids explored the surface, very little proteinaceous residue remains at the contact points, as shown by the few, dull-reflective spots (arrowed). On mOEG, the spots only persisted for as long as the cyprid remained in contact with the surface implying that, on detachment, the protein remained on the antennules. The scale bars in each frame are 100 μm. Reproduced with permission from ref. 28 , © 2008 American Vacuum Society. Full size image Two general (non-exclusive) strategies are typically followed in the design of novel, non-biocidal, non-fouling surfaces. In this review, we distinguish between AF coatings, in which the objective is to deter the recruitment stages of fouling organisms from attaching in the first place, and 'fouling-release' (FR) coatings, which do not prevent organisms from attaching, but the interfacial bond is weakened so that attached organisms are more easily removed by the hydrodynamic shear forces generated by movement of the ship through the water [29] or by gentle 'grooming' devices [30] . In both cases the objective is to achieve the desired result through manipulation of the physico-chemical and/or materials properties of the coating (for example, elastic modulus, frictional coefficient) so that the organism either perceives the surface as unconducive to settlement or the intermolecular interaction forces between the surface and the polymeric adhesives produced by the fouling organism are weakened, promoting adhesive failure. These two general approaches are not mutually exclusive and in fact the distinction is overly simplistic. Most current commercial FR coatings are based on poly(dimethylsiloxane) elastomers (PDMSe) [31] . These non-polar, low surface energy ( ∼ 22 mN m −1 ), hydrophobic polymers would be expected to show low adhesion of polar molecules (including adhesive proteins) because of reduced opportunities for H-binding and polar interactions. Coatings based on PDMSe also have typically low elastic moduli, and the release of hard-fouling is proportional to ( γE ) ½ ; where γ is the surface energy and E is the modulus [32] . Although PDMSe exhibit the desired combination of low surface energy (to minimize the work of adhesion) and low modulus, such coatings suffer from some disadvantages. Because of their low surface energy, they are difficult to bond to a substrate without an appropriate tie coat. They are less durable, more easily damaged than other types of coating and they frequently 'fail' to brown slimes dominated by diatoms that attach more strongly to hydrophobic surfaces [19] , [33] . The fouling-release technology is also most effective when applied to high-activity, fast-moving (>15 knot) vessels and is less suitable for vessels that spend long periods in port or which cruise at lower speeds to maintain fuel efficiency. For these and other reasons, there has been extensive research on newer fouling-release technologies [31] , which may either 'toughen up' silicones through the use of new tie-coats and the incorporation of fluoropolymers or which seek to create a surface complexity. Currently in vogue are amphiphilic coatings, which incorporate some of the benefits of both hydrophobic and hydrophilic functionalities, for example, the latest fouling-release coating from International Paint, Intersleek 900. Such coatings, through phase separation, for example, of mutually incompatible block copolymers, create a dynamic surface with local variations in surface chemistry, topography and mechanical properties. The general aim is to create a dynamic and compositional surface complexity that deters settlement stages of fouling organisms and reduces the interfacial bonding with adhesive polymers. Here we review the range of experimental coating technologies currently being explored as the basis for future practical AF coatings. Only a few of these technologies have reached the stage of evaluation in the field, for example, as test panels on rafts, and there are no published reports of field performance. The main focus will be on polymer-based experimental systems that can be envisaged as the basis for future practical coatings for application to ship hulls. The accent will be on studies that demonstrate clear coating structure/property/performance correlations and the importance of using surface characterization techniques under in situ (that is, immersed) conditions in order to assess surface reorganization and to understand the type of surface that the settling stages (cells and larvae) encounter. The section will also consider the current interest in biomimetic/bioinspired technologies and efforts to rationalize the influence of surface roughness through predictive models. Bioinspired engineered topographies It is often observed that many marine organisms do not become colonized by other species [8] , [34] , [35] , [36] , [37] . A diverse range of mechanisms has been implicated in natural defence, including settlement-inhibiting micro- and nanotopographies, secreted bioactive molecules, sloughing surface layers, mucus secretions and hydrolytic enzymes (see ref. 38 for review). Natural mechanisms may be used as the basis for 'biomimetic' or 'bioinspired' coatings, and most attention has been devoted to designs based on topographical features. The surfaces of many marine animals ranging from shells of molluscs to the skin of sharks and whales have a complex surface topography, and by analogy with the 'self-cleaning' lotus-leaf effect, it is often speculated that this surface roughness may have a role in either deterring fouling organisms from attaching or promoting their easy release. These thoughts have encouraged research on a number of bioinspired surface designs [35] of which the most prominent for marine applications are those that mimic sharkskin [39] and invertebrate shells [40] . Moulded topographies in PDMSe ( Box 1 ), inspired by the skin of fast-moving sharks at ∼ 1/25th of the scale (Sharklet AF, Fig. 5 ), resulted in an 85% reduction in settlement of zoospores (motile spores) of the macroalga Ulva compared with smooth PDMSe [39] . The Sharklet AF topography consists of 2μm wide rectangular-like (ribs) periodic features (4, 8, 12 and 16 μm in length) spaced 2 μm apart. Further studies based on 2μm features correlated zoospore settlement with an empirically derived 'engineered roughness index' (ERI I ) for various surface designs [41] , [42] . ERI I is a dimensionless ratio involving several geometric parameters of the surfaces: where r is the Wenzel's roughness factor, (1− ϕ s ) is the area fraction of feature tops (that is, the ratio of the depressed surface area between features and the projected planar surface area) and df is the degree of freedom of spore movement (1 or 2). Spore settlement decreased with an increase in ERI I . Sharklet AF with an ERI I of 9.5 showing a 77% reduction in settlement compared with the smooth surface. 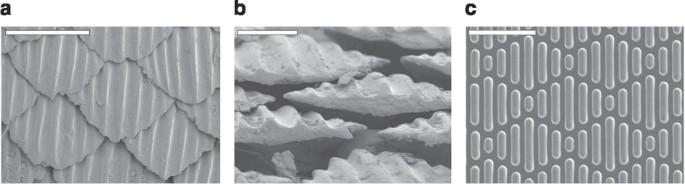Figure 5: Bioinspired topographies to deter fouling. The scanning electron micrographs show the skin denticles of spinner shark in face (a) and end (b) views and (c) image of Sharklet AF topography moulded in PDMSe. Scale bars are (a) 500 μm, (b) 250 μm and (c) 20 μm. Images courtesy of: Professor A.B. Brennan. Figure 5: Bioinspired topographies to deter fouling. The scanning electron micrographs show the skin denticles of spinner shark in face ( a ) and end ( b ) views and ( c ) image of Sharklet AF topography moulded in PDMSe. Scale bars are ( a ) 500 μm, ( b ) 250 μm and ( c ) 20 μm. Images courtesy of: Professor A.B. Brennan. Full size image Schumacher et al . [43] introduced the concept of nanoforce gradients to explain how different feature geometries based on the Sharklet design might exert an influence on the settlement of spores. It was hypothesized that nanoforce gradients caused by variations in topographical feature geometry will induce stress gradients within the lateral plane of the cell membrane of a settling cell during initial contact. Perception of such stress gradients by presumed mechanotransducer proteins in the cell membrane could, through intracellular signal cascades, lead to modification of the settlement response. The generation of the nanoforce gradients was envisaged as a function of the bending moment or stiffness of the topographical features with which the cell is in contact. The geometric dimensions, including width, length and height of the topographical feature, as well as the modulus of the base material, define its stiffness. By introducing geometric variations in features contained in the engineered topography, an effective force gradient between neighbouring topographical features is developed. To test the nanoforce gradient hypothesis, modifications were made to the design of Sharklet AF, resulting in a range of nanoforce gradients [43] . The surfaces were then challenged with spores of Ulva . Surfaces with nanoforce gradients ranging from 125 to 374 nN all significantly reduced spore settlement relative to a smooth substrate, but the level of inhibition did not correlate directly with the magnitude of the gradient, nor was the level of inhibition predicted by ERI I . It became evident that the number of distinct features was a better predictor of inhibition by the topographies and this led to substitution of d f by n , in a revised ERI model (ERI II ). Settlement densities of spores of Ulva were affected by the complexity of the microtopographical patterns, settlement decreasing as the number of features increased ( Fig. 6 ). The number of attached spores per unit area was normalized to the number of spores attached to a smooth control and the data were transformed by taking the natural logarithm (ln A / A o ). The spore settlement density on the different patterns correlated well with the number of features and the ERI (ERI II ) model [42] . Furthermore, the level of spore settlement on several novel surface designs and some designs tested previously was correctly predicted by the ERI II model [42] . 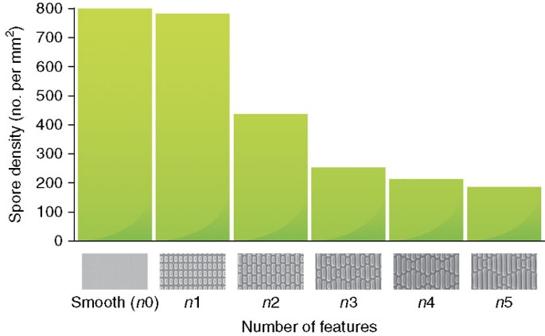Figure 6: Settlement of spores ofUlvaon microengineered Sharklet AF patterns moulded in PDMSe. The graph shows the results of an experiment in which spores ofUlvawere allowed to settle (adhere) to a variety of 'Sharklet-type' patterns, with increasing numbers of distinct topographic features. The height of the bars indicates the resulting density of spores settled on the different patterns, which are illustrated below each bar (from left to right,n=0 (smooth), 1–5, wheren=the number of distinct topographic features). In all cases, the height and spacing of the features remained constant (2.8 μm high×2 μm wide×2 μm space). Figure drawn from data in ref.42; images of patterns courtesy of Professor A.B. Brennan. Figure 6: Settlement of spores of Ulva on microengineered Sharklet AF patterns moulded in PDMSe. The graph shows the results of an experiment in which spores of Ulva were allowed to settle (adhere) to a variety of 'Sharklet-type' patterns, with increasing numbers of distinct topographic features. The height of the bars indicates the resulting density of spores settled on the different patterns, which are illustrated below each bar (from left to right, n =0 (smooth), 1–5, where n =the number of distinct topographic features). In all cases, the height and spacing of the features remained constant (2.8 μm high×2 μm wide×2 μm space). Figure drawn from data in ref. 42 ; images of patterns courtesy of Professor A.B. Brennan. Full size image These results confirm that the designed nanoforce gradients may be an effective tool and predictive model for the design of unique non-toxic, non-fouling surfaces for marine applications. However, as different fouling organisms respond to topographies of different length scales, hierarchical patterning may be required. An initial study by Schumacher et al . [44] indicated that complex designs would be required to repel multiple settling species. Current research on the 'Sharklet effect' attempts to combine topography with different chemistries at the surface or in the bulk, to further intensify the deterrent effect. It should also be pointed out that to be successful, bioinspired technologies will require multiple attributes (topography, modulus and chemistry) to be effective in the marine environment. The organisms that have provided the inspiration for this area of research, for example, mussels, use several strategies to keep themselves 'clean' [34] , and hierarchical topographic designs will be needed to combat settlement of all cells and larvae [44] . Box 1: GLOSSARY Amphiphilic: A term describing molecules or surfaces that simultaneously possess both hydrophilic and hydrophobic properties. Antifouling: As in 'antifouling coatings'—measures that prevent the colonization of immersed structures. Biofilm: An aggregate of microorganisms adhering to each other and to a surface and embedded in a slimy matrix of extracellular polymeric substances (EPS). In the context of marine fouling, a biofilm is a complex community of unicells including bacteria, diatoms and protozoa. Biofouling: The undesirable accumulation of microorganisms, seaweeds and invertebrate animals on structures immersed in aquatic environments. Fouling-release (as in 'fouling-release coatings'): refers to coatings that do not prevent colonization, but the adhering organisms are so weakly attached that they are released at low hydrodynamic shear forces, such as those created when a vessel moves through the water. Hydrophilic: Literally 'water loving', refers to the physical property of molecules or surfaces that can bond with water molecules through hydrogen bonding. This means that surface is very wettable, that is, a droplet of water readily spreads on such a surface. Hydrophobic: Literally 'water hating', refers to a physical property of molecules or surfaces that cannot readily bond with water or other polar molecules. 'Superhydrophobic' surfaces are extremely difficult to wet, that is, water droplets roll off when the surface is tilted by as little as 10° (often referred to as the 'Lotus effect'). Biocides: Chemical substances that kill organisms and are therefore widely used in medicine (e.g. bacteriocides), agriculture (pesticides and fungicides) and many areas of industry, including fouling control in which they are the active ingredients in current commercial antifouling paints. PDMSe: Poly(dimethylsiloxane) elastomer, a rubbery polymer that forms the binder system of many commercial fouling-release coatings. Zwitterion: Chemical compounds with both positive and negative charges on different atoms, and a total net charge of zero. Betaines are a specific type of zwitterions bearing a positively charged quaternary ammonium group and a negatively charged carboxylate group. Nanocomposite: A multiphase solid material in which one of the phases has a dimension of <100 nm, as, for example, the result of including nanoparticles such as nanoclay mineral particles or carbon nanotubes. Amphiphilic nanostructured coatings A recent trend in designing experimental coatings for AF/fouling-release purposes has been to create surfaces with compositional (chemical) heterogeneity at the nanoscale through the thermodynamically driven, phase segregation of polymer assemblies, followed by crosslinking in situ . These coating designs may be based on blends of immiscible polymers or contrasting chemistries of block copolymers, and the general aim is to combine the non-polar, low surface energy properties of a hydrophobic (typically fluorinated) component to reduce polar and hydrogen-bonding interactions with the bioadhesives used by fouling organisms, with the well-known protein repellency properties of the hydrophilic components, typically, oligo(poly)ethylene glycols. The resulting chemical ambiguity, expressed in terms of amphiphilic nanodomains on the surface ( Fig. 7 ), may lower the entropic and enthalpic driving forces for the adsorption of the marine protein and glycoprotein bioadhesives, which are themselves amphiphilic in character [45] , [46] . Lau et al . [47] have speculated that the often-observed protein resistance of some nanopatterned, amphiphilic diblock copolymers is due to the intrinsic high density of surface interfacial boundaries. 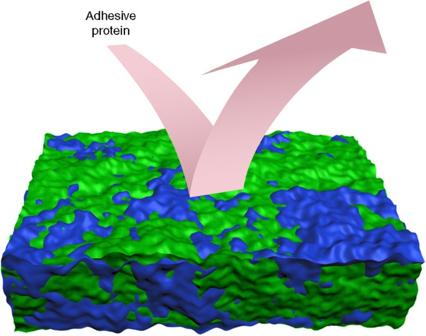Figure 7: The concept of a chemically heterogeneous or 'mosaic-like' surface that repels proteins. Such chemically 'ambiguous' coatings could be based, for example, on the combination of fluorinated, hydrophobic segments (green) and hydrophilic poly(ethyleneglycol) segments (blue), thus imparting an amphiphilic character. The relative scale of the amphiphilic patches is not intended to indicate accurate dimensions. Cartoon of amphiphilic surface courtesy of Professor Karen Wooley. Figure 7: The concept of a chemically heterogeneous or 'mosaic-like' surface that repels proteins. Such chemically 'ambiguous' coatings could be based, for example, on the combination of fluorinated, hydrophobic segments (green) and hydrophilic poly(ethyleneglycol) segments (blue), thus imparting an amphiphilic character. The relative scale of the amphiphilic patches is not intended to indicate accurate dimensions. Cartoon of amphiphilic surface courtesy of Professor Karen Wooley. Full size image The first published example of an amphiphilic coating for use in marine AF is that of ref. 48 , based on hyperbranched fluoropolymers and linear poly(ethylene glycols) (PEG), which self-assemble on cross-linking to form complex surface topographies and chemical domains of both nanoscopic and microscopic dimensions. The surface patterns were strongly influenced by immersion and by the relative proportions of the two polymers. The coating design anticipated that this surface complexity would either have a deterrent effect on the settling stages of fouling organisms or would be unfavourable for adsorption and unfolding of adhesive proteins. Gudipati et al . [49] subsequently showed that several macromolecules of biological origin (proteins and lipopolysaccharides) showed reduced adsorption to compositions with high concentrations of PEG (45–55% by weight). These compositions were also effective against settlement of zoospores of the green alga Ulva , and small plants of Ulva adhered less well to some of the compositions compared with PDMSe. Krishnan et al . [50] used side-chain grafting of hydrophilic oligoethylene glycol and hydrophobic perfluoroalkyl side chains to a preformed poly(styrene- block -acrylic acid) copolymer. Martinelli et al . [51] , [52] developed similar amphiphilic copolymers using controlled atom transfer radical polymerization and a purely polystyrene backbone. In both cases, these surface-active block copolymers were deposited as a thin film over a thick layer of SEBS (poly(styrene- block -ethylene- random -butylene)- block -polystyrene), an elastomeric thermoplastic material that provides a suitable low modulus [53] . In both studies, NEXAFS and angle-resolved X-ray photoelectron spectroscopy measurements demonstrated that the film surface underwent reconstruction resulting from the thermodynamically induced phase segregation of the mutually incompatible components. However, these are in vacuo techniques and it is difficult to translate the information they provide on surface structure in the dry state to the situation when these coatings are immersed in water. To understand the relationship between surface properties and biological performance, it is necessary to perform surface characterization in the immersed state. In situ (underwater) atomic force microscopy showed that surface topography changed on immersion, presumably caused by localized swelling of the hydrophilic blocks [51] ( Fig. 8 ). Information on the surface chemistry of immersed coatings was provided by Sum Frequency Generation spectroscopy, which showed that, in water, the hydrophilic PEG segments migrated to the surface and surprisingly the hydrophobic, fluorinated groups were still evident, suggesting that the surface is truly amphiphilic in nature [54] . These coatings have been tested in bioassays to explore their intrinsic ability to resist the settlement and reduce the adhesion strength of two marine algae, namely, the macroalga (seaweed) Ulva and the unicellular diatom Na v icula . These organisms were chosen specifically because they show opposite preferences, Ulva tends to adhere most strongly to hydrophilic coatings while diatom species such as Navicula adhere most strongly to hydrophobic coatings, especially those that are silicone-based. Both Ulva and Navicula showed weak adhesion to the amphiphilic surface-active block copolymers coatings compared with a standard fouling-release coating of PDMSe [46] , [51] . 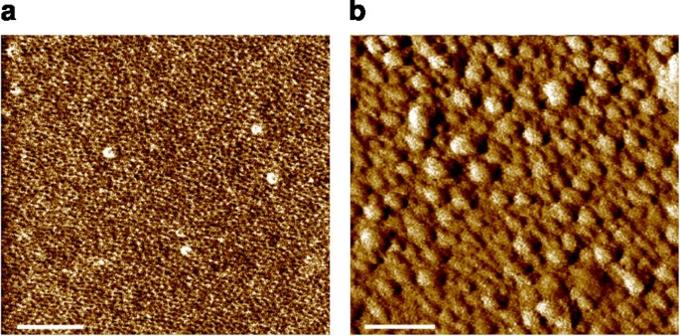Figure 8: AFM images of an amphiphilic coating showing the influence of immersion on surface nanostructure. AFM phase images of polystyrene-based amphiphilic diblock fluorinated/PEGylated copolymer coatings were obtained in tapping mode (a) before, and (b) after immersion for 7 days in artificial seawater. Scale bars are 200 nm. Images reproduced with permission from ref.51, © 2008 American Chemical Society. Figure 8: AFM images of an amphiphilic coating showing the influence of immersion on surface nanostructure. AFM phase images of polystyrene-based amphiphilic diblock fluorinated/PEGylated copolymer coatings were obtained in tapping mode ( a ) before, and ( b ) after immersion for 7 days in artificial seawater. Scale bars are 200 nm. Images reproduced with permission from ref. 51 , © 2008 American Chemical Society. Full size image Phase-segregating siloxane–polyurethane copolymers In an attempt to improve the mechanical properties of PDMS elastomers, thermosetting, cross-linked PDMSe–polyurethane nanohybrid copolymer coatings have been synthesized [55] , [56] , [57] , [58] . Certain compositions (those containing only 10% PDMSe) spontaneously phase-separated to form microtopographic domains composed of PDMSe surrounded by the polyurethane matrix. The domains appeared to increase in size after 2-week immersion: stability depended on the casting solvent [55] and mixing time [57] used. Compositions with a higher proportion of PDMSe did not form domains, but rather formed a smooth stratified coating of low surface energy PDMSe over a sub-layer of higher surface energy polyurethane. In detachment studies with 'pseudobarnacles' (an epoxy-bonded stud used as a proxy for live barnacles) and with reattached live barnacles, it was shown that the pull-off force in both cases was lower on compositions with surface domains than those without [57] . Majumdar et al . [59] investigated the AF and fouling-release properties of PDMSe with tethered quaternary ammonium salts (QAS). The initial concept was to combine the biocidal properties of QAS with the fouling-release properties of PDMSe. Surface analysis of the resultant coatings revealed a heterogeneous, two-phase morphology with increased water contact angle (increased hydrophobicity). Depending on the QAS alkyl chain length, surface protrusions were either isolated, 0.7–2.6 μm in size (C14), or inter-connected, 0.60–2.9 μm in size (C18). The C18 coatings also showed higher levels of nanoroughness. In laboratory tests with a range of fouling organisms, the rougher C18 coatings showed the best fouling-release performance against the macroalga Ulva exceeding that of a commercially available FR coating. FR performance against Ulva is unlikely to be related to the tethered biocidal functionality per se , as the coatings did not affect growth of the alga, but rather seems to be related to the nanoroughness. On the other hand, it was shown that the QAS coatings inhibited microbial biofilm formation of the bacterium Cellulophaga lytica and the diatom Navicula incerta —which is most likely due to the biocidal functionality. Superhydrophilic zwitterionic polymers The limitations in terms of stability of protein-resistant molecules such as PEG for marine applications have been referred to earlier. A more promising group of chemistries that deter the adsorption of proteins and cells are zwitterionic materials, such as poly(sulphobetaine) and poly(carboxybetaine). These materials have good chemical stability and low cost [60] . The majority of the published papers on zwitterionic coatings relate to proteins, serum or medically important bacteria (reviewed in ref. 60 ). In AF assays polySBMA brushes grafted onto glass surfaces through surface-initiated atom transfer radical polymerization almost completely inhibited the settlement of spores of the green alga Ulva and the attachment of diatom cells was also strongly reduced. In both cases, the few cells that did settle were only loosely attached [61] . Both polySBMA and polyCBMA resisted settlement of barnacle cypris larvae, but as noted above (Insights from in situ imaging of surface exploration), larval searching behaviour differed on the two zwitterionic surfaces [26] . The resistance of zwitterionic materials to the adsorption of proteins and cells is generally attributed to a strong electrostatically induced hydration layer that creates a superhydrophilic surface. In the case of marine organisms this means that the secreted proteoglycan bioadhesives are unable to achieve a strong interfacial bond by excluding water molecules from the interface. The future development of hydrolyzable zwitterionic esters as coatings should provide a platform for the development of practical marine coatings [60] . Inorganic–organic nanohybrids Organically modified, hybrid xerogel coatings prepared by the sol-gel process have been shown to possess AF and fouling-release characteristics [62] , [63] , [64] , [65] . The xerogel surfaces are inexpensive and robust, characterized by uniform surface roughness/topography and cover a range of wettabilities and surface energies. The settlement of barnacle cyprids and algal zoospores was highly correlated with surface energy and wettability, as was the removal of algal ( Ulva ) sporelings (young plants) and adhered diatoms [62] , [65] . However, the response to these surface parameters was not uniform; cypris larvae of Balanus amphitrite prefered to settle on xerogel surfaces with high wettability and high surface energy [65] , while zoospores of Ulva prefered to settle on hydrophobic xerogel surfaces with low surface energy [62] . Sporelings of Ulva were more readily removed from surfaces with low wettability and low surface energy (Bennett et al . [62] ), while diatoms were more readily removed from surfaces with high wettability and high surface energy [65] . The current xerogel formulations are only suitable for low-fouling freshwater environments in which slime predominates, as the thin ( ∼ 1 μm) xerogels do not have fouling-release properties for adult barnacles. To improve AF performance in marine environments, sequestration of catalysts, for example, diorganoselenoxides and diorganotellurides, into the xerogel films that facilitate the oxidation of halide salts with naturally occurring hydrogen peroxide to form the corresponding hypochlorous acid have shown promise against the settlement of barnacle and tubeworm larvae and algal spores [64] . Nanocomposites and superhydrophic surfaces Hydrosilation-cured silicone elastomers, reinforced through the incorporation of small quantities of multiwall carbon nanotubes (MWCNTs) and sepiolite nanoclays, showed enhanced fouling-release performance in laboratory assays with algae and barnacles compared with unfilled PDMSe controls [66] . The use of MWCNTs is particularly significant, as the improved performance was obtained at low loadings of the nanofiller (0.05–0.2% by weight). At this level of loading the bulk properties of the coatings (tensile modulus and cross-link density) appear to be unchanged, but the coatings became slightly more hydrophobic and there was a significant change in shear-thinning behaviour [67] . The changed rheological properties were attributed, on both theoretical and experimental grounds, to a strong molecular affinity between the siloxane chains and the MWCNTs, through CH-π interactions involving methyl groups of the PDMSe and aromatic rings of the MWCNTs [67] . This affinity is also important in reducing the likelihood of MWCNTs being released into the marine (or any other) environment, which is relevant to the current debate on potential issues of nanoparticle toxicity. The improved fouling-release performance appears to be correlated with the effect of MWCNTs in inducing time- and immersion-dependent changes in surface nanotopography [68] . Under tapping-mode AFM, both unfilled and MWCNT-filled PDMSe showed a smooth morphology (root mean squared (RMS) roughness ∼ 1 nm), but after immersion in water, there was a complex time-dependent surface restructuring of both filled and unfilled coatings, and those containing 0.1% MWCNTs exhibited a significant restructuring at the nanoscale. It is not yet clear how such nanostructuring contributes towards fouling-release performance. Superhydrophobic surfaces are water-repellent, having a high water contact angle (typically >150°) and a very low roll-off angle, that is, the inclination angle at which a water drop rolls off the surfaces [69] . The superhydrophobic effect relies on the trapping of air, as exemplified by a number of natural surfaces, for example, the lotus leaf and insect wings [37] . Recently, Scardino et al . [36] reported three superhydrophobic coatings (SHC) that inhibit the settlement/attachment of spores of algae and larvae of several invertebrates. The coatings were made by spraying fumed silica-filled siloxanes. All three coatings were superhydrophobic (SHC 1 contact angle θ A =169°, SHC 2 θ A =155° and SHC 3 θ A =169°) and exhibited either micro/nanoroughness (SHC 1 and 2) or only nanoroughness (SHC 3). All test organisms avoided settling on the SHC 3 coating, which had large pores of ∼ 350 nm in diameter and small pores in the range of 10–50 nm. Small-angle X-ray scattering was used to characterize the partial wetting of the superhydrophobic surfaces in situ under immersion conditions. The broad-spectrum AF effect was attributed to the larger amount of unwetted interface on SHC 3 compared with SHC 1 and 2 when immersed in seawater. Whether the unwetted interface will resist wetting (and hence the accumulation of fouling) following long-term immersion needs to be determined. Current commercial, non-biocidal fouling-release coatings, suffer from a number of drawbacks and represent only a small proportion of the total marine coatings market [31] . In the near future it is likely that coatings to combat marine biofouling will be based on what are considered to be 'eco-friendly' biocides (for example, by tethering to the coating or by using biocides with low toxicity and short half-lives) [70] . However, we have shown in this review that significant research efforts are being directed towards the discovery or improvement of novel, non-toxic, non-fouling coatings as alternatives to those currently used commercially. We have given several examples demonstrating that fouling organisms are influenced in their initial surface colonization behaviour, and the subsequent development of adhesion strength, by nano- and micro-scale-engineered coating designs. The examples chosen are not exhaustive, and there is abundant research on other ways of combating fouling organisms through non-toxic coating designs that we have not been able to discuss. For example, protein-degrading enzymes (serine proteases) have been shown to be effective in reducing settlement and adhesion strength of a range of fouling organisms, algal spores, diatoms and barnacle cyprids [71] , due to dissolution of adhesive [72] , [73] . However, the challenge for enzyme technology will be to achieve controlled release and stability of enzymes when incorporated into a coating [74] , [75] . In some cases, the novel coatings we have discussed are real candidates for practical application after further development work. However, little is known about the mechanism(s) by which these engineered coatings exert their effects. We have shown several examples of correlations between specific types of morphological or chemical surface structuring and biological performance. However, correlation does not imply causality and there are real knowledge barriers to understanding how these coatings work. Advances are needed to understand the underlying biological and molecular mechanisms. For example, there is almost no information available for the common macrofouling organisms on what the critical length scale is of the structures involved in surface sensing, nor the molecular basis of their functioning (it is presumed that similar to other cell types, spores of seaweeds, barnacle larvae etc possess mechanotransducing proteins and stretch-sensitive ion channels in their surface membranes that can sense and initiate responses to surface structures, but there are no actual reports of such proteins). We have shown in this review that there is a growing body of evidence that amphiphilic or chemically 'ambiguous' coatings present both polar and non-polar functionalities to a fouling organism and show promising performance against a wide range of fouling organisms; indeed, examples of this type of coating, such as Intersleek 900, are available commercially. However, relatively little is understood about the underlying 'design rules' or the biological basis of performance. Specifically, more understanding of coating surface properties in the immersed condition, rather than in dry or in vacuo is needed, as immersion changes the dynamics of self-assembly and surface organization. For example, in the case of coatings based on amphiphilic PEGylated and fluorinated copolymers, the hypothesis is that these are structured to present a chemically complex surface to fouling organisms. But, is the reduced adhesion observed solely due to the reduced ability of adhesive proteins to adsorb to the PEGylated domains (PEG is well known to be resistant to protein adsorption [76] ) and what are the critical dimensions of the hydrophilic/hydrophobic surface domains? Furthermore, on immersion in the natural marine environment, the surface properties of the coatings may change further due to surface conditioning by adsorption of macromolecules and microorganisms [77] , which will also vary according to season and geographic location. The development of novel, nanorough, fouling-release polysiloxanes containing carbon nanotubes is intriguing, but at present there is no understanding as to the mechanistic basis of this effect; does the nanoroughness cause the cells/larvae to adhere less strongly (that is, a 'biological' basis) or is a 'physical' mechanism more likely whereby nano- and micro-air incursions, such as those postulated for SHCs [36] , reduce the interfacial contact between adhesive and surface, thereby reducing adhesion strength? Interdisciplinary studies combining chemistry, biology and advanced physical techniques for interfacial characterization will be crucial in advancing this field. The control of biofouling of surfaces in the marine environment is a considerable challenge: the fouling organisms are opportunists and have evolved the capability to attach and proliferate on a range of surfaces in the natural, highly turbulent marine environment. We consider it unlikely that non-biocidal solutions based on coating designs incorporating a single attribute will solve the problem. One way forward will be to design 'multifunctional coatings', incorporating a range of attributes, for example, an appropriate topography combined with a suitable amphiphilic or zwitterionic surface chemistry and environmentally benign compounds that deter settlement or enzymes to target their bioadhesives. Bioinspired 'smart' coatings combining topography with sacrificial or renewable, low-fouling polymers to shed fouling organisms in a manner analogous to marine mammals [78] may emerge as a practical concept. Fortunately, there is no shortage of innovative ideas! The challenge is to persuade funding agencies that expenditure on research and development will translate into real benefits in terms of economics and reduced environmental burdens. A recent economic analysis [3] shows that a small improvement in the condition of the hulls would produce a significant saving. For example, if improved AF technology could produce just a modest reduction in overall fouling level on one class of destroyers operated by the US Navy (for example, from 'heavy slime' to 'light slime'), that alone would result in a saving of $19 M per annum! How to cite this article: Callow, J. A. & Callow, M. E. Trends in the development of environmentally friendly fouling-resistant marine coatings. Nat. Commun. 2:244 doi: 10.1038/ncomms1251 (2011).